Glia- and neuron-specific functions of TrkB signalling during retinal degeneration and regeneration Glia, the support cells of the central nervous system, have recently attracted considerable attention both as mediators of neural cell survival and as sources of neural regeneration. To further elucidate the role of glial and neural cells in neurodegeneration, we generated TrkB GFAP and TrkB c-kit knockout mice in which TrkB, a receptor for brain-derived neurotrophic factor (BDNF), is deleted in retinal glia or inner retinal neurons, respectively. Here, we show that the extent of glutamate-induced retinal degeneration was similar in these two mutant mice. Furthermore in TrkB GFAP knockout mice, BDNF did not prevent photoreceptor degeneration and failed to stimulate Müller glial cell proliferation and expression of neural markers in the degenerating retina. These results demonstrate that BDNF signalling in glia has important roles in neural protection and regeneration, particularly in conversion of Müller glia to photoreceptors. In addition, our genetic models provide a system in which glia- and neuron-specific gene functions can be tested in central nervous system tissues in vivo . In the central nervous system (CNS), glial cells have long been thought to simply provide scaffolding and physical support for neurons, whose electrical impulses underlie all sensation, movement and thought. However, recent studies have demonstrated that glia, which account for 90% of the cells in some regions of the human brain, have more significant roles than previously hypothesized [1] . For example, glial cells guide migrating neurons to their destinations, control synapse number and may participate in the homeostatic activity-dependent regulation of synaptic connectivity [2] , [3] . In addition, radial glial cells, which express a number of markers also expressed by neural progenitors, were demonstrated to dedifferentiate, proliferate and give rise to neurons in vivo [4] , [5] , [6] . We previously demonstrated that the glutamate transporter GLAST, one such progenitor marker [7] , is expressed in retina-specific Müller glial cells, which are thought to carry out many of the functions of radial glia, astrocytes and oligodendrocytes in the CNS [8] , [9] . Müller glial cells dedifferentiate in response to neurotoxic damage or injury, implying that even the adult mammalian retina may have regenerative potential [10] , [11] . The response of Müller glia to acute retinal damage may be mediated by growth factors produced by retinal cells, such as basic fibroblast growth factor (bFGF) and brain-derived neurotrophic factor (BDNF) [12] , [13] , [14] . BDNF is known to regulate neural cell survival and axonal outgrowth mainly by activating TrkB receptors, which stimulates various signalling cascades, such as mitogen-activated protein kinase pathway, phosphatidylinositol 3-kinase pathway and Fyn-mediated actin polymerization [15] , [16] , [17] . However, TrkB expression is low in photoreceptors relative to other retinal cell types, including retinal ganglion cells (RGCs) and Müller glia [12] , [13] , [18] . Consequently, we previously proposed a model in which exogenously applied or microglia-derived neurotrophins regulate photoreceptor survival indirectly by regulating secondary trophic factor production in Müller glia [12] , [19] . However, the effects that such a glia-neuron interaction would have in vivo or whether it would be relevant for the protection of neural cell types that express TrkB remained unclear. In the present study, we prepared two conditional knockout (KO) mice in which TrkB was deleted from retinal glia or from two types of retinal neurons (RGCs and amacrine cells). These mice enabled us to separately examine direct and indirect effects of TrkB on neuroprotection. We demonstrate that TrkB signalling in Müller glia is critically involved in neural protection and regeneration during retinal degeneration. These mice may enable the further study of genes involved in the glia-neuron network and neurodegeneration. Glia- and neuron-specific TrkB ablation in the retina Previous studies have shown that the GFAP -Cre transgenic strain, in which Cre expression is regulated by the human GFAP promoter, expresses Cre recombinase not only in mature astrocytes but also in multipotent radial glial cells that exhibit neural stem/progenitor cell properties [20] , [21] . To examine expression of the GFAP -Cre transgene in the adult retina, we crossed GFAP -Cre mice with a Rosa26-LacZ reporter line [22] , [23] in which recombination results in expression of β-galactosidase (β-gal; Fig. 1a,b ). To identify the specific β-gal immunopositive (IP) cell type(s), we carried out co-staining with markers of other retinal lineages. β-gal-IP cells were double labelled with glutamine synthetase (GS; a marker of Müller glial cells), but not with calretinin (a marker of RGCs and amacrine cells), calbindin (a marker of horizontal cells) or protein kinase C (PKC; a marker of bipolar cells; Fig. 1b ). These results revealed that β-gal expression, which reflects Cre recombinase expression, is restricted to glial cells in GFAP -Cre LacZ mice. On the other hand, in c-kit -Cre LacZ mice [24] , β-gal-IP cells were double labelled with calretinin and TUJ1 (another RGC marker), but not with GS, calbindin or PKC ( Fig. 1b ). These results indicate that, in contrast to GFAP -Cre LacZ mice, expression of Cre recombinase is restricted to RGCs and amacrine cells in c-kit -Cre LacZ mice ( Fig. 1a ). 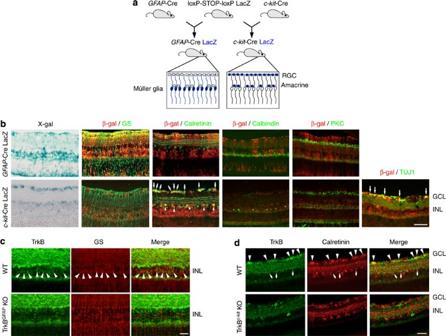Figure 1: Establishment of glia- and neuron-specific TrkB conditional KO mice. (a) Schematic diagram of transgenically targeted fate-mapping strategy.GFAP-Cre andc-kit-Cre mice were crossed with Rosa26-LacZ reporter mice. In Cre reporter offspring, only cells that express Cre excise a loxP-flanked stop signal and activate constitutive LacZ expression. Blue colour depicts LacZ-positive cells. (b) X-gal staining (blue) and immunostaining (red) of β-gal-positive cells. Glutamine synthetase (GS), calretinin, calbindin, protein kinase C (PKC) and TUJ1 were used as cell type-specific markers (green). Overlapping immunoreactivities (yellow) of β-gal and GS, calretinin or TUJ1 indicate that Cre-mediated recombination occurs in Müller glial cells inGFAP-Cre LacZ mice, and RGCs (arrows) and amacrine cells (arrowheads) inc-kit-Cre LacZ mice. (c) Immunohistochemical analysis of TrkB (green) and GS (red) showed loss of TrkB from Müller glial cells (arrowheads) in TrkBGFAPKO mice. (d) Immunohistochemical analysis of TrkB (green) and calretinin (red) showed loss of TrkB from RGCs (arrowheads) and amacrine cells (arrows) in TrkBc-kitKO mice. Scale bar, 100 μm. GCL, ganglion cell layer; INL, inner nuclear layer; RGC, retinal ganglion cell. Figure 1: Establishment of glia- and neuron-specific TrkB conditional KO mice. ( a ) Schematic diagram of transgenically targeted fate-mapping strategy. GFAP -Cre and c-kit -Cre mice were crossed with Rosa26-LacZ reporter mice. In Cre reporter offspring, only cells that express Cre excise a loxP-flanked stop signal and activate constitutive LacZ expression. Blue colour depicts LacZ-positive cells. ( b ) X-gal staining (blue) and immunostaining (red) of β-gal-positive cells. Glutamine synthetase (GS), calretinin, calbindin, protein kinase C (PKC) and TUJ1 were used as cell type-specific markers (green). Overlapping immunoreactivities (yellow) of β-gal and GS, calretinin or TUJ1 indicate that Cre-mediated recombination occurs in Müller glial cells in GFAP -Cre LacZ mice, and RGCs (arrows) and amacrine cells (arrowheads) in c-kit -Cre LacZ mice. ( c ) Immunohistochemical analysis of TrkB (green) and GS (red) showed loss of TrkB from Müller glial cells (arrowheads) in TrkB GFAP KO mice. ( d ) Immunohistochemical analysis of TrkB (green) and calretinin (red) showed loss of TrkB from RGCs (arrowheads) and amacrine cells (arrows) in TrkB c-kit KO mice. Scale bar, 100 μm. GCL, ganglion cell layer; INL, inner nuclear layer; RGC, retinal ganglion cell. Full size image To selectively eliminate TrkB from retinal glia or neurons, we next crossed TrkB flox/flox mice [25] with GFAP -Cre or c-kit -Cre mice. The resulting double transgenic TrkB flox/flox ; GFAP -Cre+ and TrkB flox/flox ; c-kit -Cre+ mice were termed as TrkB GFAP KO mice and TrkB c-kit KO mice, respectively. Retinal development and structure were normal in both strains compared with wild-type (WT) mice ( Supplementary Fig. S1 ). Immunohistochemical analysis revealed that TrkB protein expression in Müller glia (arrowheads in Fig. 1c ) was eliminated in TrkB GFAP KO mice. In contrast, TrkB expression was eliminated in RGCs (arrowheads in Fig. 1d ) and amacrine cells (arrows in Fig. 1d ) in TrkB c-kit KO mice. Taken together, these findings demonstrate that GFAP -Cre and c-kit -Cre virtually eliminated TrkB expression from retinal glia and neurons, respectively. Direct and indirect effects of BDNF on RGC protection Neurotrophins prevent RGC death from glutamate neurotoxicity [26] . As RGCs express TrkB receptors, we compared the roles of TrkB signalling in RGCs and Müller glia in BDNF-dependent neuroprotection to determine the direct and indirect effects, respectively. For this purpose, we prepared retinal explants from WT, TrkB c-kit KO and TrkB GFAP KO mice ( Fig. 2a ). The WT retinal explants stimulated with 5 mM glutamate for 1 h showed a decrease in the number of NeuN-positive neurons in the ganglion cell layer (GCL) compared with the untreated control explants ( Fig. 2a,b ). As expected, the same treatment significantly decreased the number of surviving RGCs in the TrkB c-kit KO mouse retina. We predicted milder RGC degeneration in the TrkB GFAP KO compared with the TrkB c-kit KO mouse retina; however, RGC loss was as severe as that observed in the TrkB c-kit KO mouse retina ( Fig. 2a,b ). These results suggest that, at least under our experimental conditions, the indirect protective effect of BDNF by Müller glia is as powerful as the direct effect through TrkB in RGCs. 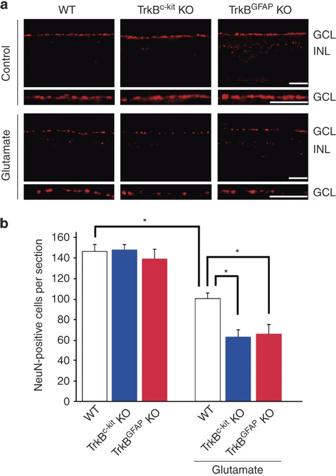Figure 2: Similar susceptibility to glutamate neurotoxicity in TrkBc-kitKO and TrkBGFAPKO retinas. (a) Immunohistochemical analysis of mouse retinal explants from WT, TrkBc-kitKO and TrkBGFAPKO mice stained with an anti-NeuN antibody. Explants were untreated (control) or treated with 5 mM glutamate for 1 h. Scale bar, 50 μm. (b) Quantification of NeuN-positive cells in the GCL. Data are shown as the mean+s.e.m. (n=6). *P<0.01. GCL, ganglion cell layer; INL, inner nuclear layer. Figure 2: Similar susceptibility to glutamate neurotoxicity in TrkB c-kit KO and TrkB GFAP KO retinas. ( a ) Immunohistochemical analysis of mouse retinal explants from WT, TrkB c-kit KO and TrkB GFAP KO mice stained with an anti-NeuN antibody. Explants were untreated (control) or treated with 5 mM glutamate for 1 h. Scale bar, 50 μm. ( b ) Quantification of NeuN-positive cells in the GCL. Data are shown as the mean+s.e.m. ( n =6). * P <0.01. GCL, ganglion cell layer; INL, inner nuclear layer. Full size image To further examine the function of TrkB signalling in retinal glia, we next prepared cultured Müller cells from WT and TrkB GFAP KO mice and analysed them by western blot. Consistent with the immunohistochemical results ( Fig. 1c ), TrkB protein expression in Müller glia was not detectable in TrkB GFAP KO mice ( Fig. 3a ). We next examined whether exogenous BDNF stimulates TrkB-dependent signal transduction in Müller glia by observing the activation of cyclic AMP response element-binding (CREB) protein. In WT Müller cells, the basal phosphorylated CREB (pCREB) expression level was very low, but BDNF clearly increased the ratio of pCREB to CREB ( Fig. 3b ). In contrast, the effect of BDNF on CREB activation was only marginal in TrkB GFAP KO Müller cells ( Fig. 3b ). We also examined the effect of BDNF on CREB phosphorylation in vivo . In WT retinas, intraocular injection of BDNF induced pCREB expression in RGCs and Müller glia (arrow and arrowhead in Fig. 3c ). In TrkB GFAP KO mice, BDNF-induced pCREB expression in RGCs was comparable with WT retinas, but expression was barely detectable in Müller glia ( Fig. 3c ). These results confirmed a lack of TrkB-dependent signal transduction in Müller glia in TrkB GFAP KO mice. We previously demonstrated that treatment of cultured rat Müller cells with BDNF increases the production of several trophic factors that can protect retinal neurons [19] . Similarly, in mouse Müller cells, BDNF increased mRNA expression levels of BDNF, bFGF, ciliary neurotrophic factor and glial cell line-derived neurotrophic factor ( Fig. 3d ). However, BDNF failed to stimulate the production of trophic factors in Müller cells prepared from TrkB GFAP KO mice ( Fig. 3d ). Thus, TrkB elimination in Müller glia impairs the transcription of trophic factors, which may lead to RGC vulnerability during glutamate neurotoxicity. 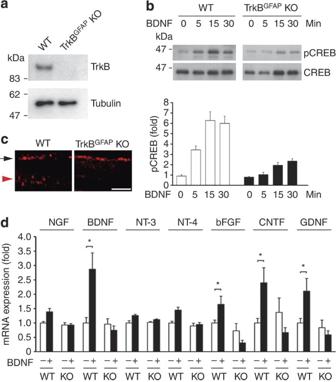Figure 3: Functional analysis of Müller glial cells in TrkBGFAPKO mice. (a) Immunoblot analysis of TrkB protein in cultured Müller cells from WT and TrkBGFAPKO mice. (b) Immunoblot analysis of phosphorylated CREB (pCREB) and total CREB in cultured Müller cells from WT and TrkBGFAPKO mice. BDNF (50 ng ml−1)-induced CREB phosphorylation was impaired in TrkBGFAPKO Müller cells. For each determination, the ratio of pCREB/CREB protein level in controls (WT, BDNF 0 min) was normalized to a value of 1.0. Data are shown as the mean+s.e.m. (n=3). (c) Immunohistochemical analysis of pCREB in BDNF (1 μg μl−1)-treated WT and TrkBGFAPKO retinas. Note the absence of pCREB in Müller cells (red arrowhead) of the TrkBGFAPKO retina, despite its persistence in the GCL (arrow). Scale bar, 50 μm. (d) Effect of BDNF (100 ng ml−1for 48 h) on trophic factor production in cultured Müller cells from WT and TrkBGFAPKO mice. For each determination, the mRNA level in controls (WT, without BDNF) was normalized to a value of 1.0. Data are shown as the mean+s.e.m. (n=6). *P<0.05. NGF, nerve growth factor; NT-3, neurotrophin-3; NT-4, neurotrophin-4; CNTF, ciliary neurotrophic factor; GNDF, glial cell line-derived neurotrophic factor. Figure 3: Functional analysis of Müller glial cells in TrkB GFAP KO mice. ( a ) Immunoblot analysis of TrkB protein in cultured Müller cells from WT and TrkB GFAP KO mice. ( b ) Immunoblot analysis of phosphorylated CREB (pCREB) and total CREB in cultured Müller cells from WT and TrkB GFAP KO mice. BDNF (50 ng ml −1 )-induced CREB phosphorylation was impaired in TrkB GFAP KO Müller cells. For each determination, the ratio of pCREB/CREB protein level in controls (WT, BDNF 0 min) was normalized to a value of 1.0. Data are shown as the mean+s.e.m. ( n =3). ( c ) Immunohistochemical analysis of pCREB in BDNF (1 μg μl −1 )-treated WT and TrkB GFAP KO retinas. Note the absence of pCREB in Müller cells (red arrowhead) of the TrkB GFAP KO retina, despite its persistence in the GCL (arrow). Scale bar, 50 μm. ( d ) Effect of BDNF (100 ng ml −1 for 48 h) on trophic factor production in cultured Müller cells from WT and TrkB GFAP KO mice. For each determination, the mRNA level in controls (WT, without BDNF) was normalized to a value of 1.0. Data are shown as the mean+s.e.m. ( n =6). * P <0.05. NGF, nerve growth factor; NT-3, neurotrophin-3; NT-4, neurotrophin-4; CNTF, ciliary neurotrophic factor; GNDF, glial cell line-derived neurotrophic factor. Full size image Accelerated photoreceptor degeneration in TrkB GFAP KO Various trophic factors rescue photoreceptors during retinal degeneration [27] , [28] , [29] . As photoreceptors do not express a high level of neurotrophin receptors, the indirect glia-mediated rescue pathway may be more important for photoreceptors than for other cell types, including RGCs [12] , [13] , [18] . To further elucidate the effect of the glia-neuron network in neuroprotection in vivo , we used a second animal disease model, N -methyl- N -nitrosourea (MNU)-induced photoreceptor degeneration ( Fig. 4a ). MNU is an alkylating agent that causes DNA methylation and activates caspases, leading to photoreceptor apoptosis in various animal species [30] . In WT mice, 15 mg kg −1 MNU decreased the thickness of the outer nuclear layer (ONL), but intravitreous injection of BDNF partially rescued the photoreceptor loss ( Fig. 4b,c ). However, in TrkB GFAP KO mice, 7.5 mg kg −1 MNU resulted in an ∼ 50% loss of the ONL, which was significantly greater than the loss in WT retinas, and BDNF failed to induce photoreceptor survival against any doses of MNU ( Fig. 4b,c ). The protective effect of BDNF in WT mice diminished in the presence of a higher dose of MNU (60 mg kg −1 ); this dose completely abolished the ONL but left the inner retinal layer (IRL) intact ( Fig. 4b,d ). In contrast, the same dose of MNU applied to TrkB GFAP KO mice induced considerable loss of the IRL as well as the removal of the ONL ( Fig. 4b,d ). These in vivo data suggest that glial TrkB signalling has a pivotal role in the protection of surrounding neurons. 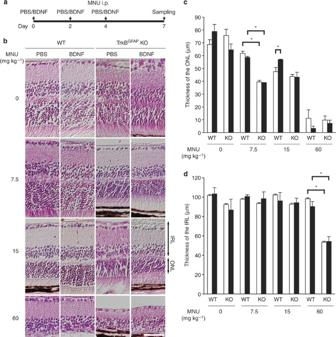Figure 4: Accelerated photoreceptor degeneration in TrkBGFAPKO mice. (a) Animal protocols for MNU-induced photoreceptor degeneration. MNU was injected intraperitoneally (i.p.) into WT and TrkBGFAPKO mice at the concentration of 0, 7.5, 15 or 60 mg kg−1. PBS or BDNF (1 μg μl−1) was intraocularly injected at day 0, 2 and 4, and the animals were killed at day 7 after MNU treatment. (b) Representative photomicrographs of PBS- or BDNF-treated retinas from WT and TrkBGFAPKO mice administered with various concentrations of MNU. Scale bar, 50 μm. (c,d) Quantitative analysis of the thickness of the ONL (c) and the IRL (d) in PBS (white bar)- or BDNF (black bar)-treated retinas. Data are shown as the mean s.e.m. (n=4). *P<0.05. IRL, inner retinal layer; ONL, outer nuclear layer. Figure 4: Accelerated photoreceptor degeneration in TrkB GFAP KO mice. ( a ) Animal protocols for MNU-induced photoreceptor degeneration. MNU was injected intraperitoneally (i.p.) into WT and TrkB GFAP KO mice at the concentration of 0, 7.5, 15 or 60 mg kg −1 . PBS or BDNF (1 μg μl −1 ) was intraocularly injected at day 0, 2 and 4, and the animals were killed at day 7 after MNU treatment. ( b ) Representative photomicrographs of PBS- or BDNF-treated retinas from WT and TrkB GFAP KO mice administered with various concentrations of MNU. Scale bar, 50 μm. ( c , d ) Quantitative analysis of the thickness of the ONL ( c ) and the IRL ( d ) in PBS (white bar)- or BDNF (black bar)-treated retinas. Data are shown as the mean s.e.m. ( n =4). * P <0.05. IRL, inner retinal layer; ONL, outer nuclear layer. Full size image Regenerative capacity of Müller glia through TrkB signalling Recent studies have provided evidence that radial glia sustain neural regeneration even in the adult brain [4] , [5] , [6] . Müller glia are considered to be a type of radial glia that may function as retinal progenitor cells [10] , [11] . We therefore examined the regenerative response of Müller cells to BDNF in the MNU-induced photoreceptor degeneration model ( Fig. 5a ). To observe dividing cells, we labelled WT and TrkB GFAP KO animals with 5-bromodeoxyuridin (BrdU). Although few BrdU-labelled cells were detected at day 5, intraocular injection of BDNF clearly increased BrdU-labelling in GLAST-IP cells in the inner retina (arrows) and in some cells in the ONL ( Fig. 5b ). In contrast, BDNF injection did not promote BrdU incorporation in TrkB GFAP KO mice or WT mice treated with K252a, an inhibitor of Trk receptors ( Fig. 5b ). At day 7, BDNF-induced BrdU-positive cells were detected predominantly in the remaining ONL, where they were co-labelled with rod photoreceptor markers, such as rhodopsin and recoverin ( Fig. 5c ). However, BDNF-induced BrdU incorporation was suppressed in TrkB GFAP KO mice ( Supplementary Fig. S2 ). Furthermore, these BrdU-labelled cells were overlapped with β-gal staining in GFAP -Cre LacZ mice, providing evidence that they were derived from Müller glia ( Fig. 5c ). In addition, some BrdU-positive cells were detected in the inner retina and double labelled with Brn3b (another RGC marker) or calretinin ( Fig. 5d ). These results suggest the possibility that BDNF can convert the proliferating Müller glia to rod photoreceptors and, to a lesser extent, to other retinal neurons in the MNU model. Thus, TrkB deficiency achieved by Cre-mediated recombination results in the loss of regenerating Müller cells. 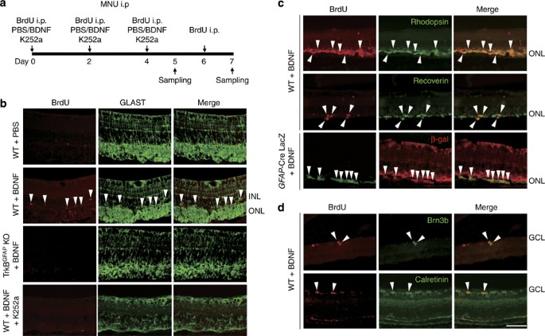Figure 5: Effect of BDNF on the proliferation of Müller glial cells during retinal degeneration. (a) Animal protocols. MNU (60 mg kg−1) was injected intraperitoneally (i.p.) to WT, TrkBGFAPKO andGFAP-Cre LacZ mice. BrdU (50 mg kg−1) was injected (i.p.) at day 0, 2, 4 and 6 after MNU treatment. PBS, BDNF (1 μg μl−1) and K252a (1 mM) were intraocularly injected at day 0, 2 and 4, and the animals were killed at day 5 or 7. (b) Sections of the retina treated with PBS, BDNF and K252a in WT and TrkBGFAPKO mice (day 5). BDNF increased BrdU-labelling in GLAST-positive cells in the INL (arrowheads) and some cells in the ONL in WT, but not in TrkBGFAPKO mice. K252a (a blocker for Trk receptors) inhibited BDNF-induced BrdU expression. (c) BrdU-labelled cells in the ONL were double labelled (arrowheads) with rhodopsin or recoverin in WT mice, and with β-gal inGFAP-Cre LacZ mice (day 7). (d) BrdU-labelled cells in the GCL were double labelled (arrowheads) with Brn3b or calretinin (day 7). Scale bar, 50 μm. GCL, ganglion cell layer; INL, inner nuclear layer; ONL, outer nuclear layer. Figure 5: Effect of BDNF on the proliferation of Müller glial cells during retinal degeneration. ( a ) Animal protocols. MNU (60 mg kg −1 ) was injected intraperitoneally (i.p.) to WT, TrkB GFAP KO and GFAP -Cre LacZ mice. BrdU (50 mg kg −1 ) was injected (i.p.) at day 0, 2, 4 and 6 after MNU treatment. PBS, BDNF (1 μg μl −1 ) and K252a (1 mM) were intraocularly injected at day 0, 2 and 4, and the animals were killed at day 5 or 7. ( b ) Sections of the retina treated with PBS, BDNF and K252a in WT and TrkB GFAP KO mice (day 5). BDNF increased BrdU-labelling in GLAST-positive cells in the INL (arrowheads) and some cells in the ONL in WT, but not in TrkB GFAP KO mice. K252a (a blocker for Trk receptors) inhibited BDNF-induced BrdU expression. ( c ) BrdU-labelled cells in the ONL were double labelled (arrowheads) with rhodopsin or recoverin in WT mice, and with β-gal in GFAP -Cre LacZ mice (day 7). ( d ) BrdU-labelled cells in the GCL were double labelled (arrowheads) with Brn3b or calretinin (day 7). Scale bar, 50 μm. GCL, ganglion cell layer; INL, inner nuclear layer; ONL, outer nuclear layer. Full size image We further examined the effects of BDNF on cultured Müller cells and found increased nestin expression, a neural stem/progenitor cell marker, in WT but not in TrkB GFAP KO Müller cells ( Fig. 6a ). When neural stem cells are induced to differentiate into the neurogenic pathway, Mash1 , a proneural gene, is derepressed through a signalling cascade that depends on expression of the calcium/calmodulin-dependent protein kinase IIδ (CaMKIIδ) [31] , [32] . In the retina, Mash1 is involved in the generation of bipolar cells and photoreceptors from progenitor cells [33] , [34] . A previous study showed that CaMKIIδ mediates the phosphorylation of Hes1, which is required for Mash1 activation [31] . As BDNF can stimulate CaMKII through TrkB [16] , we next examined whether BDNF regulates this pathway in neural regeneration. We found that BDNF increased Mash1 levels in WT but not in TrkB GFAP KO Müller cells, and the subsequent quantitative analysis revealed that BDNF had no effect on Hes1 expression ( Fig. 6b,c ). In addition, BDNF significantly increased the expression level of CaMKIIδ but not CaMKIIα, CaMKIIβ or CaMKIIγ in WT Müller cells ( Fig. 6d ). The BDNF-induced increase of CaMKIIδ was not detected in TrkB GFAP KO Müller cells ( Fig. 6d ). In contrast, platelet-derived growth factor, which can also activate CaMKII (ref. 31 ), increased nestin and Mash1 expression in both WT and TrkB GFAP KO Müller cells ( Fig. 6e,f ). These results suggest that BDNF signalling through TrkB stimulates the CaMKIIδ-Mash1 pathway, which induces the potential capacity of Müller glia as intrinsic retinal progenitor cells. 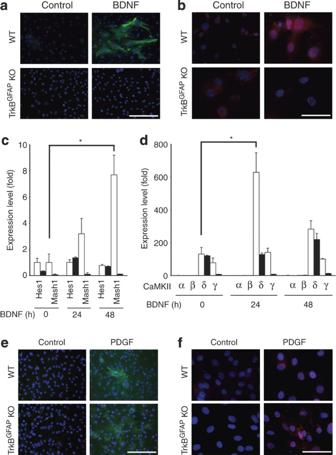Figure 6: Regenerative capacity of Müller glial cells mediated by TrkB signalling. (a,b) Treatment with BDNF (100 ng ml−1for 1–2 days) induced expression of nestin (a) and Mash1 (b) in cultured Müller cells from WT but not TrkBGFAPKO mice. (c,d) Expression of Hes1 and Mash1 (c) and CaMKII (d) in BDNF-treated Müller cells from WT (white bar) and TrkBGFAPKO (black bar) mice. Note the upregulation of CaMKIIδ and Mash1 in WT but not TrkBGFAPKO Müller cells. Data are shown as the mean+s.e.m. (n=4). *P<0.01. (e,f) Treatment with platelet-derived growth factor (PDGF; 50 ng ml−1for 24 h) induced expression of nestin (e) and Mash1 (f) in cultured Müller cells from WT and TrkBGFAPKO mice. Scale bars, 150 μm (a,e) and 50 μm (b,f). Figure 6: Regenerative capacity of Müller glial cells mediated by TrkB signalling. ( a , b ) Treatment with BDNF (100 ng ml −1 for 1–2 days) induced expression of nestin ( a ) and Mash1 ( b ) in cultured Müller cells from WT but not TrkB GFAP KO mice. ( c , d ) Expression of Hes1 and Mash1 ( c ) and CaMKII ( d ) in BDNF-treated Müller cells from WT (white bar) and TrkB GFAP KO (black bar) mice. Note the upregulation of CaMKIIδ and Mash1 in WT but not TrkB GFAP KO Müller cells. Data are shown as the mean+s.e.m. ( n =4). * P <0.01. ( e , f ) Treatment with platelet-derived growth factor (PDGF; 50 ng ml −1 for 24 h) induced expression of nestin ( e ) and Mash1 ( f ) in cultured Müller cells from WT and TrkB GFAP KO mice. Scale bars, 150 μm ( a , e ) and 50 μm ( b , f ). Full size image In the present study, we used TrkB GFAP and TrkB c-kit KO mice to explore TrkB functions in retinal Müller glia and inner retinal neurons, respectively. We observed that the extent of glutamate-induced retinal degeneration was almost equal in these two mutant mouse models. In addition, BDNF failed to prevent photoreceptor degeneration in TrkB GFAP KO mice. These findings represent the first direct evidence for a role of neurotrophin receptors in glial cells during retinal degeneration. Our results are consistent with the previous assumption that the glia-neuron network is heavily involved in the protection of surrounding neurons in vivo [12] , [13] , [14] , [19] . Another intriguing result is that BDNF–TrkB signalling stimulated Müller cells to proliferate and express retinal neural cell markers. This finding supports previous work, suggesting that Müller cells have regenerative potential [10] , [11] . Thus, both BDNF stimulation and intrinsic signal transduction through TrkB may be required for Müller glia to become endogenous retinal progenitor cells. As BDNF induces the production of various trophic factors in Müller cells, including bFGF and insulin growth factor, the regeneration process may involve these trophic factors by an autocrine process. Taken together, our results suggest that neurotrophin signalling in glia is an important mediator of neuroprotection as well as a signalling cue to induce regeneration of radial glia in vivo . In the retina, glutamate excitotoxicity and oxidative stress may contribute to various eye diseases, including retinal ischaemia and glaucoma [8] , [9] , [35] , [36] , [37] , [38] . In these disorders, loss of RGCs and subsequent optic nerve degeneration are the primary concerns. As RGCs express Trk receptors, neurotrophins are thought to directly regulate RGC number during development and prevent RGC death in the adult retina [34] . However, our results suggest an unexpectedly powerful neuroprotective effect of TrkB signalling in Müller glia. One possible explanation for this phenomenon is that the total neuroprotective effect of Müller glia-derived trophic factors ( Fig. 3d ) is as effective as that of direct BDNF signalling in RGCs ( Fig. 2 ) (ref. 39 ). Consistently, transcorneal electrical stimulation, which stimulates Müller cell production of insulin growth factor-1 and BDNF, rescues axotomized RGCs and improves retinal function in human patients [40] , [41] . Although the number is small compared with Müller glia, we cannot exclude the possibility that astrocytes located in the GCL may also be involved in RGC rescue. Compared with RGC degeneration, photoreceptor degeneration is a relatively simple disease model in which to explore TrkB function, because TrkB expression is low in photoreceptors [12] , [13] , [18] . In the present study, using the TrkB GFAP KO mouse, we demonstrated a functional glia-neuron network during photoreceptor degeneration in vivo . As BDNF increases ciliary neurotrophic factor and glial cell line-derived neurotrophic factor production in WT, but not in TrkB-deficient Müller cells ( Fig. 3d ), which can directly protect photoreceptors as well as RGCs [12] , [19] , [27] , BDNF seems to exert photoreceptor protection by a paracrine mechanism. Consistently, MNU-induced photoreceptor degeneration was observed at a lower dose in TrkB GFAP KO mice compared with WT mice, and BDNF failed to prevent or delay the degeneration process in the mutant ( Fig. 4 ). Moreover, we found that MNU induced unusual thinning of IRLs in TrkB GFAP KO animals ( Fig. 4 ). These results again suggest the importance of glial TrkB signalling for the protection of various types of surrounding neurons during retinal degeneration. One may find that the protective effects of exogenous BDNF observed in our study are small. As our MNU model is a relatively acute model, it is possible that exogenous BDNF may be more effective in other models that represent milder, slow-progressive photoreceptor degeneration. We also examined the effect of BDNF on Müller glial cells as intrinsic retinal progenitor cells. We found that BDNF–TrkB signalling stimulated the CaMKIIδ-Mash1 pathway and induced the expression of rod photoreceptor markers in proliferating Müller cells ( Figs 5 and 6 ). This finding is consistent with the previous work that Mash1 is involved in the generation of photoreceptors from retinal progenitor cells [33] , [34] . A recent study demonstrated that exogenous Wnt3a increases the proliferation of Müller cells in the photoreceptor-damaged adult mouse retina [42] . As Wnt modulates CaMK activity [43] , Wnt signalling may promote adult neurogenesis, at least partly, through the CaMKIIδ-Mash1 pathway. In fact, CaMKII activation restored the regeneration capability in the TrkB-deficient Müller cells ( Fig. 6e,f ). CaMK is a calcium-dependent kinase and activation of CaMK can in turn lead to phosphorylation of CREB [44] . In our TrkB GFAP KO mice, BDNF-induced CREB phosphorylation was almost absent in Müller cells, whereas it was clearly detectable in RGCs ( Fig. 3c ). In astrocytes, TrkB-T1, a truncated form of TrkB that lacks tyrosine kinase activity, may mediate calcium signalling [45] . However, both full-length and truncated forms of TrkB are deleted in our TrkB GFAP KO mice [25] , and thus, we have not been able to determine which form of TrkB is necessary for the proliferation and differentiation of Müller cells. Further investigation into subtype-specific TrkB functions in Müller cells may lead to the identification of relevant secondary trophic factors and mechanisms of effective regeneration in the degenerating retina. We also showed that BDNF induces the expression of RGC markers in proliferating, that is, BrdU-positive, cells in MNU-treated mice ( Fig. 5 ). However, the rate of occurrence and the number of identified cells were much lower than those for photoreceptor markers. It is possible that degenerating photoreceptors in MNU-treated mice may release trophic factors [46] , including bFGF, which could act in combination with BDNF to stimulate Müller cell proliferation in the ONL. However, this study clearly demonstrates that BDNF–TrkB signalling is one of the active pathways involved in Müller glial cell regeneration. Additional RGC degeneration models and further TrkB signalling and effector pathway studies may lead to better understanding of the mechanisms and transcriptional regulators at play. In summary, we report important roles of neurotrophin signalling in glial cells as well as in neural cells. Loss of TrkB signalling in glial cells led to severe retinal degeneration in two different animal models. In addition, BDNF–TrkB signalling stimulated the proliferation and differentiation of dedifferentiated Müller glial cells in the degenerating retina. Our glia- and neuron-specific KO mice offer a powerful system for investigating region-specific functions of target genes as well as their contributions to the glia-neuron network in vivo . Recent studies have shown that the unprocessed precursor forms of neurotrophin family members, for example, proBDNF, are released from neurons during development and in adulthood, and such molecules can act through a co-receptor system of p75 NTR and sortilin [47] , [48] . Thus, further study is required to determine whether Müller glia-derived BDNF includes proBDNF and, if so, whether proBDNF induces neural cell apoptosis or inhibits the regenerative potential of Müller cells in vivo . Mice Experiments were performed using TrkB flox/flox ; GFAP- Cre+ (TrkB GFAP KO) and TrkB flox/flox ; c-kit -Cre+ (TrkB c-kit KO) mice [22] , [24] , [25] in accordance with the Tokyo Metropolitan Institute for Neuroscience Guidelines for the Care and Use of Animals. Light intensity inside the cages ranged from 100 to 200 lux under a 12 h light/12 h dark cycle. Histological and morphometric studies Paraffin sections (7 μm thick) were cut through the optic nerve and stained with hematoxylin and eosin. The sections were examined with a Microscope (BX51; Olympus) equipped with Plan Fluor objectives connected to a DP70 camera (Olympus). The number of cells in the GCL was counted from one ora serrata through the optic nerve to the other ora serrata [37] . The thickness of the ONL and IRL (between the internal limiting membrane and the interface of the outer plexiform layer and INL) was measured using NIH Image (ImageJ 1.38) (ref. 12 ). Immunohistochemistry was performed using a Rabbit antibody against TrkB (1:200, Santa Cruz) and a Mouse antibody against GS (1:500, Chemicon) or Calretinin (1:500, Chemicon). β-gal expression in GFAP -Cre LacZ and c-kit -Cre LacZ mice Frozen retinal sections were incubated in X-gal solution at 37 °C for 12 h (ref. 23 ). For double-labelling immunohistochemistry, the sections were incubated with a Goat polyclonal antibody against β-gal (1:1,000, Biogenesis) and a Mouse antibody against GS (1:500, Chemicon), Calretinin (1:500, Chemicon), PKC (1:500, Sigma), Calbindin (1:100, Sigma) or TUJ1 (1:100, R&D). Retinal explant culture The neural retina without pigment epithelium was placed on a Millicell chamber filter (30-mm diameter, pore size 0.4 mm; Millipore) with the GCL upwards. The chambers were transferred to a 6-well culture plate, with each well containing 1 ml of DMEM/F-12 (Invitrogen) containing 20% Heat-inactivated horse serum (Invitrogen), changed every other day. The cells were cultured at 34 °C in 5% CO 2 . Retinal explant cultures were incubated with or without 5 mM glutamate for 1 h. After 72 h, retinal explants were immunostained with Mouse anti-NeuN (1:1,000, Chemicon), and the number of NeuN-positive cells in the GCL was quantified [49] . Müller cell proliferation during photoreceptor degeneration MNU was injected intraperitoneally (i.p.) into WT, TrkB GFAP KO and GFAP -Cre LacZ mice at the concentration of 7.5, 15 or 60 mg kg −1 . BrdU was injected (i.p.) at a dose of 50 mg kg −1 at day 0, 2, 4 and 6 after MNU treatment. BDNF (1 μg μl −1 ) and K252a (1 mM, Alomone Labs) were intraocularly injected at day 0, 2 and 4. At day 5 or 7, the animals were killed, and retinal sections were stained with Mouse anti-BrdU (1:20, Roche) and Rabbit anti-GLAST (1:1,000) [8] , Rabbit anti-Recoverin (1:1,000, Millipore), Goat anti-β-gal (1:1,000, Biogenesis) or Goat anti-Brn3b (1:200, Santa Cruz) antibodies. Some sections were stained with Rat anti-BrdU (1:40, Abcam) and Mouse anti-Rhodopsin (1:1,000, Sigma) or Mouse anti-Calretinin (1:500, Chemicon) antibodies. The number of BrdU-positive or BrdU/rhodopsin-double positive cells was counted from one ora serrata through the optic nerve to the other ora serrata [37] . Müller cell culture Primary Müller cells [19] were treated with 50 ng ml −1 of BDNF for 0–0.5, 12 or 24 h, and 50 ng ml −1 of platelet-derived growth factor for 24 h. Immunocytochemical analysis was performed with Mouse anti-Nestin (1:100, Chemicon) and Rabbit anti-Mash1 (1:40, R&D) antibodies, followed by 4,6-diamidino-2-phenylindole staining. Total RNA was extracted with Isogen (Nippon Gene) according to the manufacturer's protocol. Resultant RNA was treated with DNase (RQ1 RNase-Free DNase; Promega) and reverse-transcribed with Revertra ace (Toyobo) to obtain cDNA. Quantitative reverse transcription PCR was performed using the ABI 7500 fast real-time PCR system with SYBR Green PCR Master Mix (Applied Biosystems) [50] . Thermo cycling of each reaction was performed with each primer at a concentration of 100 nM. The following protocol was used: denaturation programme (95 °C for 3 min), followed by the amplification and quantification programme (95 °C for 15 s and 60 °C for 30 s) repeated for 50 cycles. The PCR quality and specificity were verified by melting curve analysis. A standard curve of cycle thresholds using serial dilutions of cDNA samples were used to calculate the relative abundance. The difference in the initial amount of total RNA between the samples was normalized in every assay using glyceraldehyde-3-phosphate dehydrogenase ( GAPDH ) gene expression as an internal standard. The primer probe pairs used are listed in Supplementary Table S1 . Immunoblotting Cultured Müller cells were homogenized in ice-cold 50 mM Tris-HCl (pH 7.4) containing 150 mM NaCl, 0.1% Triton X-100 and a protease inhibitor cocktail (Roche). Protein concentrations were determined using a Bio-Rad protein assay kit (Bio-Rad). Samples were separated on SDS polyacrylamide gel electrophoresis gels and subsequently electrotransferred to Immobilon-P filter (Millipore). Membranes were incubated with Rabbit antibodies against TrkB (1:200, Santa Cruz), Tubulin (1:1,000, Cell Signaling), CREB (1:1,000, Cell Signaling) or pCREB (1:1,000, Cell Signaling). Primary antibody binding was detected using horseradish peroxidase-labelled anti-Mouse IgG secondary antibody (Amersham) and visualized using ECL Plus western blotting system (Amersham). Statistical analyses Data are presented as means±s.e.m. For statistical analyses, a two-tailed Student's t -test was used. P <0.05 was regarded as statistically significant. How to cite this article: Harada, C. et al . Glia- and neuron-specific functions of TrkB signalling during retinal degeneration and regeneration. Nat. Commun. 2:189 doi: 10.1038/ncomms1190 (2011).